Critical role for syndecan-4 in dendritic cell migration during development of allergic airway inflammation Syndecan-4 (SDC4), expressed on dendritic cells (DCs) and activated T cells, plays a crucial role in DC motility and has been shown as a potential target for activated T-cell-driven diseases. In the present study, we investigate the role of SDC4 in the development of T-helper 2 cell-mediated allergic asthma. Using SDC4-deficient mice or an anti-SDC4 antibody we show that the absence or blocking of SDC4 signalling in ovalbumin-sensitized mice results in a reduced asthma phenotype compared with control animals. Most importantly, even established asthma is significantly decreased using the anti-SDC4 antibody. The disturbed SDC4 signalling leads to an impaired motility and directional migration of antigen-presenting DCs and therefore, to a modified sensitization leading to diminished airway inflammation. Our results demonstrate that SDC4 plays an important role in asthma induction and indicate SDC4 as possible target for therapeutic intervention in this disease. Asthma is an inappropriate T-helper 2 (Th2) cell-mediated immune response to harmless allergens and is characterized by airway inflammation, airway hyperreactivity (AHR) and increased serum immunoglobulin E (IgE) levels [1] . The initiation of a Th2-skewed immune response is dependent on signals delivered by dendritic cells (DCs), which capture and process the antigen, migrate to lymphoid organs and activate naive CD4 T cells via the T-cell receptor and accessory molecules [2] . The interaction of accessory molecules, in particular of T-cell costimulatory receptors with their ligands on antigen-presenting cells (APCs) such as DCs, is required for optimal T-cell activation. It has also been reported that accessory molecules initially described as adhesion molecules such as intercellular adhesion molecule-1 (ICAM-1) or syndecans (SDCs) may be involved in costimulatory signalling [3] , [4] . SDCs are transmembrane heparan sulfate proteoglycans interacting with growth factors and cytokines and a variety of extracellular matrix molecules via their heparan sulfate chains [5] . While SDC4 is ubiquitously expressed at low levels, an activation-dependent upregulation of SDC4 has been reported for macrophages, DCs and CD4 + T cells [6] , [7] , [8] . SDC4 expression is often involved in migration and adhesion of various cells including DCs [9] , [10] , [11] . Previous animal studies have shown a pivotal role for SDC4 in protecting against kidney injury [12] , limiting endotoxin shock [7] and promoting wound healing [13] . However, an inhibition of SDC4 by a specific antibody protected mice from cartilage damage in a murine model of osteoarthritis [14] . Moreover, the depletion of SDC4 + T cells markedly suppressed contact hypersensitivity (CHS) responses in hapten-sensitized mice [4] . Since SDC4 participates in DC migration [11] and acts as an accessory molecule during T-cell activation [4] , the aim of the current study was to examine an involvement of SDC4 in the development of a Th2-driven allergic immune response using SDC4-deficient mice. Moreover, we blocked SDC4 signalling in antigen-sensitized mice by a specific anti-SDC4 antibody not only during priming but also after an asthma-like phenotype was already established. The findings reported here clearly demonstrate a role of SDC4 in the development of allergic asthma and indicate that this molecule might be a therapeutic target for the treatment of allergic inflammatory diseases. Loss of SDC4 signalling leads to reduced allergic asthma First, the role of SDC4 in allergic asthma was investigated by comparing SDC4 −/− versus wild-type (WT) mice in a murine asthma model [15] , [16] , [17] . Histological analysis of haematoxylin and eosin (H&E)-stained lung sections showed less inflammatory infiltrates in the airways of OVA-immunized SDC4 −/− mice compared with WT animals ( Fig. 1a ) and was confirmed by an investigator-independent software based on morphometric image analysis of lung sections ( Fig. 1b ). Moreover, the total cell number in the bronchoalveolar lavage (BAL) fluid revealed a significantly decreased number of eosinophilic granulocytes in OVA-immunized SDC4 −/− mice compared with WT animals ( Fig. 1c ). In addition, the allergen-specific IgE serum levels in OVA-immunized mice were significantly lower in SDC4 −/− mice ( Fig. 1d ), as well as IgG 1 serum levels were reduced (IgG 1 titer; OVA WT: 55,138±15,886; OVA SDC4 −/− : 19,486±8,921). Accordingly, airway AHR measured as lung resistance was diminished in OVA-immunized SDC4 −/− mice compared with WT animals ( Fig. 1e ). The reduced airway inflammation and IgE serum levels in SDC4 −/− mice were associated with a drastic decreased production of the Th2 cytokines interleukin (IL)-5 and IL-13 in OVA-stimulated mediastinal lymph node cells, whereas the levels of these cytokines were unaffected in cell culture supernatants of OVA-stimulated splenocytes ( Fig. 1f,g ). The elevated cytokine levels in Alum-treated SDC4 −/− splenocytes compared with WT Alum is caused by the adjuvant since naive SDC4 −/− splenocytes did not show increased cytokine levels ( Fig. 1f ). 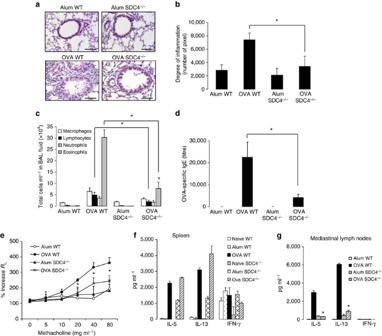Figure 1: Absence of SDC4 leads to reduced allergic immune response in OVA-immunized mice. Airway inflammation examined by (a) lung histology (H&E, × 100), (b) quantified by an investigator-independent computer-based analysis, (c) total cell number in BAL fluid, (d) OVA-specific IgE levels, (e) lung resistance and (f) cytokine production in splenocytes and (g) lymph node cells of OVA-immunized SDC4−/−mice is shown in comparison with WT control mice. Data are expressed as mean±s.e.m.,n⩾9 animals per group; *P<0.05, Student’s unpairedt-test (a–d,f,g) and one-way analysis of variance and Bonferroni’s multiple comparison test (e). Scale bars, 100 μm. Figure 1: Absence of SDC4 leads to reduced allergic immune response in OVA-immunized mice. Airway inflammation examined by ( a ) lung histology (H&E, × 100), ( b ) quantified by an investigator-independent computer-based analysis, ( c ) total cell number in BAL fluid, ( d ) OVA-specific IgE levels, ( e ) lung resistance and ( f ) cytokine production in splenocytes and ( g ) lymph node cells of OVA-immunized SDC4 −/− mice is shown in comparison with WT control mice. Data are expressed as mean±s.e.m., n ⩾ 9 animals per group; * P <0.05, Student’s unpaired t -test ( a – d , f , g ) and one-way analysis of variance and Bonferroni’s multiple comparison test ( e ). Scale bars, 100 μm. Full size image To further investigate the significance of our findings in SDC4 −/− mice (on C57BL/6 background), we inhibited SDC4 function in OVA-immunized BALB/c mice (a more Th2-dominant mouse strain) by using a polyclonal antibody that has been shown to inhibit SDC4 signalling effectively [14] . Anti-SDC4 Ab was applied on day 0 and on day 13, 1 day before OVA immunization, respectively. Anti-SDC4 Ab treatment was able to reduce the development of airway inflammation in OVA-immunized mice, as demonstrated by computer-based analysis of H&E-stained lung sections ( Fig. 2a ) and by the decreased number of eosinophils in the BAL fluid compared with control mice ( Fig. 2b ). In contrast, OVA-specific IgE serum levels were only slightly but significantly inhibited by application of anti-SDC4 Ab ( Fig. 2c ) compared with OVA-immunized mice that received only the control Ab. However, injection of anti-SDC4 Ab before immunization with OVA completely prevented the development of AHR in BALB/c mice, as demonstrated by a reduced lung resistance ( Fig. 2d ) compared with control animals. Similar to the results seen in SDC4 −/− mice, the production of IL-13 and IL-5 in OVA-stimulated splenocytes was unaffected and slightly but significantly decreased in lymph node cells by anti-SDC4 Ab ( Fig. 2e,f ). Interestingly, the levels of interferon (IFN)-γ were increased in both, spleen and mediastinal lymph nodes after anti-SDC4 treatment of OVA-immunized BALB/c mice ( Fig. 2e,f ). 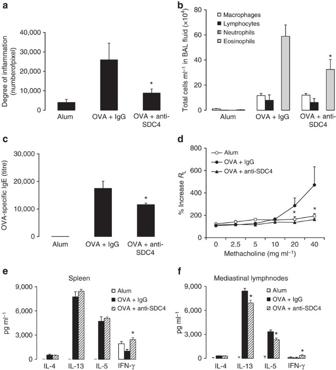Figure 2: Inhibition of SDC4 signalling by anti-SDC4 Ab during sensitization decreases the development of allergic airway inflammation. Effect of anti-SDC4 Ab treatment on days 0 and 13 one day before OVA immunization, respectively, (a) on airway inflammation, (b) the number of eosinophils in the BAL fluid, (c) OVA-specific IgE serum levels, (d) lung resistance and (e) cytokine production in splenocytes and (f) lymph node cells. Data are expressed as mean±s.e.m.,n⩾9 animals per group; *P<0.05, Student’s unpairedt-test (a–c,e,f) and one-way analysis of variance and Bonferroni’s multiple comparison test (d). Figure 2: Inhibition of SDC4 signalling by anti-SDC4 Ab during sensitization decreases the development of allergic airway inflammation. Effect of anti-SDC4 Ab treatment on days 0 and 13 one day before OVA immunization, respectively, ( a ) on airway inflammation, ( b ) the number of eosinophils in the BAL fluid, ( c ) OVA-specific IgE serum levels, ( d ) lung resistance and ( e ) cytokine production in splenocytes and ( f ) lymph node cells. Data are expressed as mean±s.e.m., n ⩾ 9 animals per group; * P <0.05, Student’s unpaired t -test ( a – c , e , f ) and one-way analysis of variance and Bonferroni’s multiple comparison test ( d ). Full size image Anti-SDC4 Ab decreased an established asthma To test the therapeutic potential of an anti-SDC4 Ab treatment during an ongoing allergic inflammation, we immunized BALB/c mice with OVA first and injected the anti-SDC4 Ab after an asthma phenotype was already fully established, similar as described before [15] . Treatment of OVA-immunized mice with anti-SDC4 Ab clearly reduced inflammation in the lung ( Fig. 3a ), the number of eosinophils in the BAL fluid ( Fig. 3b ) and OVA-specific IgE serum levels ( Fig. 3c ) compared with control Ab-treated mice. In addition, lung resistance was decreased in OVA-immunized mice that received anti-SDC4 Ab ( Fig. 3d ). Furthermore, the inhibition of IL-5 and IL-13 cytokine production in the mediastinal lymph nodes was even more distinct in the therapeutic than in the preventive approach with anti-SDC4 Ab application before OVA immunization ( Fig. 3f ). In both protocols Th2 cytokine levels in the spleen were unaffected ( Fig. 3e ). In contrast to the preventive approach, anti-SDC4 Ab treatment during an ongoing allergic inflammation had no effect on IFN-γ levels in both, lymph nodes and splenocytes ( Fig. 3e,f ). 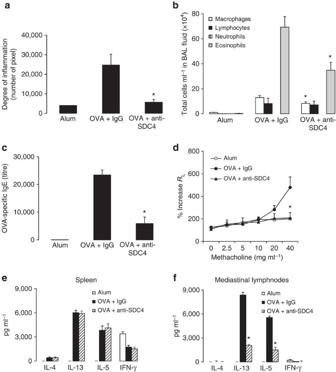Figure 3: Therapeutic effect of anti-SDC4 Ab on an established asthma phenotype. BALB/c mice were immunized with OVA on day 1 and challenged with OVA intranasally on days 14–16. Mice received the anti-SDC4 Ab or control Ab on days 18 and 22 and were challenged again with OVA on days 21–23. Effect of anti-SDC4 Ab treatment on (a) airway inflammation, (b) the number of eosinophils in the BAL fluid, (c) OVA-specific IgE serum levels, (d) lung resistance and (e) cytokine production in splenocytes and (f) lymph node cells are shown. Data are expressed as mean±s.e.m.,n⩾9 animals per group; *P<0.05, Student’s unpairedt-test (a–c,e,f) and one-way analysis of variance and Bonferroni’s multiple comparison test (d). Figure 3: Therapeutic effect of anti-SDC4 Ab on an established asthma phenotype. BALB/c mice were immunized with OVA on day 1 and challenged with OVA intranasally on days 14–16. Mice received the anti-SDC4 Ab or control Ab on days 18 and 22 and were challenged again with OVA on days 21–23. Effect of anti-SDC4 Ab treatment on ( a ) airway inflammation, ( b ) the number of eosinophils in the BAL fluid, ( c ) OVA-specific IgE serum levels, ( d ) lung resistance and ( e ) cytokine production in splenocytes and ( f ) lymph node cells are shown. Data are expressed as mean±s.e.m., n ⩾ 9 animals per group; * P <0.05, Student’s unpaired t -test ( a – c , e , f ) and one-way analysis of variance and Bonferroni’s multiple comparison test ( d ). Full size image Absence of SDC4 leads to an impaired DC motility in vivo Recently, it has been shown that SDC4 plays a crucial role in the motility of DCs [11] . Since most antigen transport in the lung is DC mediated [18] , we have investigated whether a modified DC function could be responsible for the reduced allergic immune response in the absence of SDC4. Therefore, we pulsed bone-marrow-derived DCs from SDC4 −/− or WT mice with Alexa 647-labelled OVA, stained the cells with 5-carboxy-fluoresceindiacetate (CFDA) and transferred 2 × 10 6 cells into the trachea of naive WT or SDC4 −/− mice. After OVA challenge on days 3 and 4, mediastinal lymph nodes were isolated on day 5 and CD11c + OVA-Alexa 647 + CFDA + cells were measured by flow cytometry to detect antigen-loaded DCs. In WT mice that received OVA-pulsed DCs from SDC4 −/− mice, we found less antigen-loaded CFDA + DCs than in WT or SDC4 −/− mice transferred with DCs from WT control animals ( Fig. 4a ), while the expression of certain costimulatory and adhesion molecules was comparable between WT and SDC4 −/− DCs ( Fig. 4b ). Thus, the impaired motility of SDC4 −/− DCs could result in a diminished ability to activate T cells. To investigate the consequences of a reduced appearance of APCs in the mediastinal lymph nodes for allergic inflammation in the lung, we immunized WT or SDC4 −/− mice by intrapulmonary transfer of unlabelled OVA-pulsed DCs from WT or SDC4 −/− mice-derived bone marrow, challenged mice from day 10 onwards with OVA intranasally (i.n.) for 3 consecutive days and killed animals on day 14. WT mice receiving OVA-pulsed DCs from SDC4 −/− mice showed significant less inflammation in the lung, a reduced number of eosinophils in the BAL fluid and a decreased production of IL-5 and IL-13 in the supernatant of OVA-restimulated lymph node cells compared with WT or SDC4 −/− mice treated with antigen-loaded DCs from WT animals ( Fig. 4c–e ). 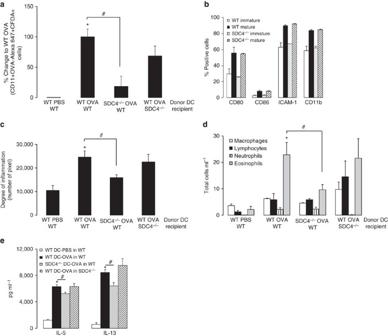Figure 4: Absence of SDC4 leads to an impaired migration of OVA-presenting DCs and to a reduced airway inflammation. Bone marrow-DCs derived from SDC4−/−or WT mice were pulsed with OVA-Alexa 647, stained with CFDA and intratracheally transferred into SDC4−/−or WT recipients. Mice were challenged with OVA on days 3 and 4 after transfer and mediastinal lymph nodes were isolated on day 5. At this time point, 0.15% cells in the lymph node were CD11+OVA-Alexa647+CFDA+. (a) Flow cytometric analysis of CD11c+OVA-Alexa 647+CFDA+cells was performed after transfer of SDC4−/−-DCs into WT recipients compared with WT mice that received WT-DCs. (b) The expression of costimulatory and adhesion molecules on mature bone-marrow-derived DCs from SDC4−/−mice in comparison with WT mice was evaluated. After transfer of unlabelled OVA-pulsed SDC4−/−-DCs and OVA challenge on days 10–12, the effect on (c) airway inflammation, (d) the number of eosinophils in the BAL fluid and (e) cytokine production in lymph node cells is shown. Data are expressed as mean±s.e.m.,n⩾7 animals per group; *P<0.05 for transfer of PBS-treated WT DCs into WT mice versus OVA-pulsed WT DCs into WT mice,#P<0.05 for OVA-pulsed WT DCs into WT mice versus OVA-pulsed SDC4−/−DCs into WT mice, Student’s unpairedt-test. Figure 4: Absence of SDC4 leads to an impaired migration of OVA-presenting DCs and to a reduced airway inflammation. Bone marrow-DCs derived from SDC4 −/− or WT mice were pulsed with OVA-Alexa 647, stained with CFDA and intratracheally transferred into SDC4 −/− or WT recipients. Mice were challenged with OVA on days 3 and 4 after transfer and mediastinal lymph nodes were isolated on day 5. At this time point, 0.15% cells in the lymph node were CD11 + OVA-Alexa647 + CFDA + . ( a ) Flow cytometric analysis of CD11c + OVA-Alexa 647 + CFDA + cells was performed after transfer of SDC4 −/− -DCs into WT recipients compared with WT mice that received WT-DCs. ( b ) The expression of costimulatory and adhesion molecules on mature bone-marrow-derived DCs from SDC4 −/− mice in comparison with WT mice was evaluated. After transfer of unlabelled OVA-pulsed SDC4 −/− -DCs and OVA challenge on days 10–12, the effect on ( c ) airway inflammation, ( d ) the number of eosinophils in the BAL fluid and ( e ) cytokine production in lymph node cells is shown. Data are expressed as mean±s.e.m., n ⩾ 7 animals per group; * P <0.05 for transfer of PBS-treated WT DCs into WT mice versus OVA-pulsed WT DCs into WT mice, # P <0.05 for OVA-pulsed WT DCs into WT mice versus OVA-pulsed SDC4 −/− DCs into WT mice, Student’s unpaired t -test. Full size image Disturbed SDC4 signalling influences directional DC migration The chemokine receptor 7 (CCR7), which is upregulated during maturation, and its ligands CCL19 and CCL21 play an important role in DC migration [19] , [20] . To evaluate directional DC migration, WT and SDC4 −/− DCs were stimulated with lipopolysaccharides (LPS), and migration towards CCL19 and CCL21 was analysed. The migration rate of SDC4-deficient DCs was significantly reduced compared with WT DCs ( Fig. 5a ). To investigate whether there is a direct interaction between these chemokines and SDC4, we performed a co-immunoprecipitation for CCL21 with flag-tagged SDC4. The data indicate that CCL21 indeed binds to SDC4, as there was only a weak binding of CCL21 detected to non-transfected HEK cells ( Fig. 5b ). 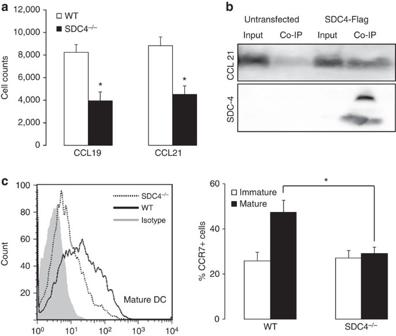Figure 5: Disturbed SDC4 signalling reduces directional DC migration and interferes with CCR7 expression. (a) The CCL19- and CCL21-directed migration in DCs from SDC4−/−mice compared with WT DCs was measured. (b) Co-immunoprecipitation (Co-IP) of CCL21 with SDC4-Flag-transfected HEK cells was performed. Untransfected HEK cells served as negative control. The presence of CCL21 was analysed by western blot in cell supernatant (input) and eluate of the Co-IP in cell supernatant (input) of both untransfected and SDC4-Flag. (c) CCR7 expression of mature BMDCs generated from SDC4−/−mice in comparison with WT DC was evaluated. Data are expressed as mean±s.e.m. of three independent experiments; *P<0.05 (a,c), Student’s unpairedt-test. (b) A representative blot of three independent experiments. Figure 5: Disturbed SDC4 signalling reduces directional DC migration and interferes with CCR7 expression. ( a ) The CCL19- and CCL21-directed migration in DCs from SDC4 −/− mice compared with WT DCs was measured. ( b ) Co-immunoprecipitation (Co-IP) of CCL21 with SDC4-Flag-transfected HEK cells was performed. Untransfected HEK cells served as negative control. The presence of CCL21 was analysed by western blot in cell supernatant (input) and eluate of the Co-IP in cell supernatant (input) of both untransfected and SDC4-Flag. ( c ) CCR7 expression of mature BMDCs generated from SDC4 −/− mice in comparison with WT DC was evaluated. Data are expressed as mean±s.e.m. of three independent experiments; * P <0.05 ( a , c ), Student’s unpaired t -test. ( b ) A representative blot of three independent experiments. Full size image As SDC4 is known to be able to influence the surface presentation of integrins by controlling the recycling of these proteins [21] , the CCR7 surface expression was analysed by flow cytometry. These investigations revealed a lower CCR7 expression on mature bone-marrow-derived dendritic cells (BMDCs) generated from SDC4 −/− mice compared with WT DCs ( Fig. 5c ). Impaired DC motility leads to a reduced CD4 + T-cell activity It has recently been shown that SDC4, which is also expressed on activated T cells, may serve as target to treat T-cell-driven diseases [4] . Using a CHS model Akiyoshi et al . [4] demonstrated that SDC4 + T cells were mainly effector memory T cells. In our model, we found an increased SDC4 expression on CD4 + T cells in the lung of OVA-immunized mice with a comparable effector memory phenotype expressing CD44 and CD45RB ( Fig. 6a ). To investigate whether SDC4 has a direct impact on activation of CD4 + T cells with consequences for the development of an allergic airway inflammation, we treated BALB/c mice with anti-SDC4 Ab or control Ab after OVA immunization. CD4 + T cells from mediastinal lymph nodes were isolated from these animals, stained with CFDA and co-cultured with irradiated splenocytes in the presence of OVA. Antigen-stimulated CD4 + T cells from OVA-immunized BALB/c mice did strongly proliferate, while the proliferation of CD4 + T cells derived from anti-SDC4 Ab-treated OVA-immunized animals was significantly reduced ( Fig. 6b ). Moreover, in this co-culture the Th2 cytokines IL-5 and IL-13 were significantly decreased in supernatants of OVA-stimulated CD4 + T cells from lymph nodes of anti-SDC4 Ab-treated OVA-immunized mice compared with control mice ( Fig. 6c ). Notably, anti-SDC4 Ab treatment of an established asthma neither depleted SDC4 + T cells in spleen, lymph nodes or lung nor SDC4 + DCs in spleen and lung. In contrast, a slightly but not significantly reduced number of SDC4 + DCs was found in the lymph nodes ( Fig. 6d ). Furthermore, in vitro co-culture of OVA-pulsed DCs with T cells carrying a transgenic OVA-recognizing T-cell receptor in the presence of anti-SDC4 Ab had no effect on CD4 + T-cell proliferation and cytokine production ( Fig. 6e,f ). 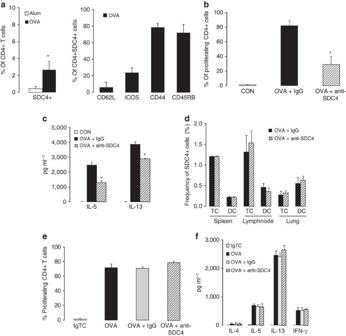Figure 6: Anti-SDC4 Ab suppresses CD4+T-cell activity. (a) SDC4 expression and specific T-cell marker were measured on separated lung CD4+T cells of OVA-immunized BALB/c mice. To analyse the role of T cells, BALB/c mice were immunized on day 1 and treated with anti-SDC4 Ab on days 3 and 7. Mice were challenged i.n. with OVA on days 6–8. CD4+T cells from mediastinal lymph nodes were isolated, stained with CFDA and co-cultured with irradiated splenocytes from BALB/c mice in the presence of OVA. (b) Proliferation and (c) cytokine production of CD4+T cells derived from anti-SDC4 Ab-treated OVA-immunized animals was measured and compared with mice treated with control Ab. (d) The frequency of SDC4+CD11c+DC and SDC4+CD4+T cells in spleen, lymph node or lung after anti-SDC4 Ab treatment was characterized. OVA-pulsed bone-marrow-derived DCs and CD4+T cells carrying a transgenic T-cell receptor for OVA were co-cultured in the presence of anti-SDC4 Ab (10 μg ml−1) for 4 days. Effect of blocking SDC4 on (e) T-cell proliferation and (f) cytokine production is shown. Data are expressed as mean±s.e.m. of three independent experiments; *P<0.05; (a) OVA versus Alum, (b,c) OVA+anti-SDC4 versus OVA+IgG, Student’s unpairedt-test. Figure 6: Anti-SDC4 Ab suppresses CD4 + T-cell activity. ( a ) SDC4 expression and specific T-cell marker were measured on separated lung CD4 + T cells of OVA-immunized BALB/c mice. To analyse the role of T cells, BALB/c mice were immunized on day 1 and treated with anti-SDC4 Ab on days 3 and 7. Mice were challenged i.n. with OVA on days 6–8. CD4 + T cells from mediastinal lymph nodes were isolated, stained with CFDA and co-cultured with irradiated splenocytes from BALB/c mice in the presence of OVA. ( b ) Proliferation and ( c ) cytokine production of CD4 + T cells derived from anti-SDC4 Ab-treated OVA-immunized animals was measured and compared with mice treated with control Ab. ( d ) The frequency of SDC4 + CD11c + DC and SDC4 + CD4 + T cells in spleen, lymph node or lung after anti-SDC4 Ab treatment was characterized. OVA-pulsed bone-marrow-derived DCs and CD4 + T cells carrying a transgenic T-cell receptor for OVA were co-cultured in the presence of anti-SDC4 Ab (10 μg ml −1 ) for 4 days. Effect of blocking SDC4 on ( e ) T-cell proliferation and ( f ) cytokine production is shown. Data are expressed as mean±s.e.m. of three independent experiments; * P <0.05; ( a ) OVA versus Alum, ( b,c ) OVA+anti-SDC4 versus OVA+IgG, Student’s unpaired t -test. Full size image Anti-SDC4 Ab treatment decreases B-cell migration Beside DCs and T cells, SDC4 might also be expressed on B cells [22] . The analysis of lymphocytes in the mediastinal lymph nodes revealed a slightly but not significantly reduced number of CD19 + and SDC4 expression on CD19 + B cells in anti-SDC4-treated mice ( Fig. 7a ). Nevertheless, we evaluated the effect of anti-SDC4 Ab treatment on B-cell function. Our results demonstrate that anti-SDC4 Ab had neither an impact on B-cell activation nor on IgE or IgG1 production ( Fig. 7b,c ). However, the CCL19-directed B-cell migration was significantly diminished after treatment with anti-SDC4 Ab ( Fig. 7d ). 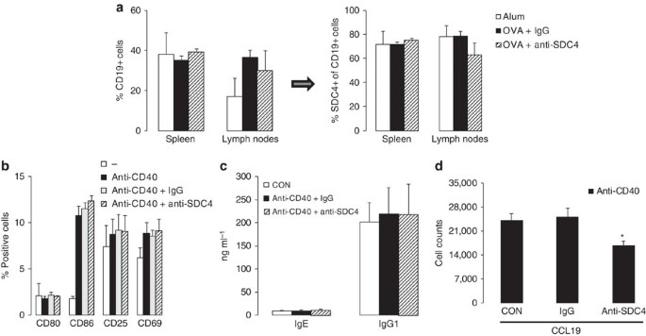Figure 7: Anti-SDC4 Ab decreases directed migration of B cells. To analyse the role of B cells, BALB/c mice were immunized on day 1 and challenged with OVA intranasally on days 14–16. Mice received the anti-SDC4 Ab or control Ab on days 18 and 22 and were challenged again with OVA on days 21–23. The effect of anti-SDC4 treatment on the frequency of CD19+B cells in lymph node and spleen and the SDC4 expression on B cells (a) is shown. Splenic CD19+B cells were isolated by magnetic-activated cell sorting andin vitroactivated with anti-CD40 (10 μg ml−1). The effect of co-incubation with anti-SDC4 Ab (10 μg ml−1) on the expression of activation and maturation marker (b) the production of IgE and IgG1antibodies (c) and the directed migration towards CCL19 (d) is demonstrated. Data are expressed as mean±s.e.m.,n⩾6 (a) orn=3 (b–d) animals per group; *P<0.05, Student’s unpairedt-test. Figure 7: Anti-SDC4 Ab decreases directed migration of B cells. To analyse the role of B cells, BALB/c mice were immunized on day 1 and challenged with OVA intranasally on days 14–16. Mice received the anti-SDC4 Ab or control Ab on days 18 and 22 and were challenged again with OVA on days 21–23. The effect of anti-SDC4 treatment on the frequency of CD19 + B cells in lymph node and spleen and the SDC4 expression on B cells ( a ) is shown. Splenic CD19 + B cells were isolated by magnetic-activated cell sorting and in vitro activated with anti-CD40 (10 μg ml −1 ). The effect of co-incubation with anti-SDC4 Ab (10 μg ml −1 ) on the expression of activation and maturation marker ( b ) the production of IgE and IgG 1 antibodies ( c ) and the directed migration towards CCL19 ( d ) is demonstrated. Data are expressed as mean±s.e.m., n ⩾ 6 ( a ) or n =3 ( b – d ) animals per group; * P <0.05, Student’s unpaired t -test. Full size image Recent findings about the role of SDC4 in DC motility and during activated T-cell-driven diseases raised the question whether SDC4 is involved in the development of an allergic immune response. Using SDC4 −/− mice and an antibody that inhibits SDC4 signalling, we could demonstrate in our established murine asthma model that absence or blocking of SDC4 signalling before the first antigen sensitization significantly reduced eosinophilic airway inflammation. Moreover, SDC4 signalling was critical for AHR development and IgE production in both, OVA-sensitized SDC4 −/− and anti-SDC4 Ab-treated mice. Furthermore, we observed a SDC4-dependent reduction of Th2 cytokine levels in mediastinal lymph nodes but not in OVA-restimulated splenocytes. These results suggest a more localized effect of SDC4, for example, by a reduced number of APCs within the inflamed tissue. It has been shown before that modulation of an asthma phenotype may result in reduced cytokine production in local lymph nodes or lung, whereas the systemic cytokine response remained unchanged [23] , [24] . The difference between the remarkably reduced inflammation/lung resistance and the moderately decreased Th2 cytokine levels in lymph nodes after anti-SDC4 Ab application might be due to the fact that, at the time of killing the Ab-mediated reduction of Th2 cell activity in the lymph nodes is already decreased, while the effect on lung inflammation and lung function persisted longer. Application of anti-SDC4 Ab shortly before killing led to a comparable decrease in lung inflammation and Th2 cytokine production in lymph nodes as shown in the therapeutic approach. However, the decreased activation of T cells in the airways might also lead to the observed diminished IgE levels. Nevertheless, the data clearly indicate a crucial role for SDC4 in the development of an allergic asthma. In contrast, the family member SDC1 seems to attenuate allergic lung inflammation as SDC1 −/− mice exhibited an exaggerated airway inflammation in a previous study [25] , whereas no information is known about an involvement of SDC2 or SDC3. The initiation of an allergic immune response is dependent on signals delivered from APCs, which capture and process the antigen and migrate to lymphoid organs to present the antigen to naive CD4 T cells [2] . Since most antigen transport into the lung is DC mediated [18] , we compared WT DCs with DCs lacking SDC4. We found a diminished number of CD11c + OVA-Alexa 647 + CFDA + cells in the mediastinal lymph nodes after adoptive transfer of DCs derived from the bone marrow from SDC4 −/− into WT recipients. The impaired migration of DCs and the missing antigen transport could be one reason for the observed reduced asthma development in SDC4 −/− mice, as the limited number of antigen-loaded DCs might result in a decreased T-cell activation. Indeed, inhibition of the accumulation of antigen-presenting DCs in the draining lymph nodes has previously been shown to reduce allergic airway inflammation [26] . Furthermore, the expression of SDC4 on DCs seems to be crucial for migration since OVA-pulsed WT DCs did migrate to the mediastinal lymph nodes in SDC4 −/− mice. An essential role for directional migration of DCs from the peripheral tissue to the draining lymph nodes was described for the chemokine receptor CCR7 and its ligands CCL19 and CCL21 (ref. 27 ). While the expression of costimulatory molecules such as CD80 or CD86 and adhesion molecules such as ICAM-1 or CD11b were comparable in WT and SDC4 −/− mice, we found that a disturbed SDC4 signalling resulted in a diminished CCR7 expression on DCs and in a reduced directional DC migration. Notably, we and others have demonstrated that some chemokines, for example, CCL21, can bind to heparan sulfate proteoglycans that may lead to changes in the sensitivity to the chemokine [28] , [29] . The absence of SDC4 on DCs may interfere with this chemokine sequestration and might explain the impaired migration of SDC4-deficient DCs to the draining lymph nodes. Moreover, it has been described that in fibroblasts lacking SDC4, migration is perturbed due to a constitutive activation of Rac and subsequent unspecific adhesion to fibronectin [30] . It is of note that Rho and Rac also control the organization of DCs’ cytoskeleton and their capacity to migrate and activate T cells [31] , [32] . A refractive activation of small RhoGTPases following CCL21 stimulation in mature SDC4 −/− DCs might hint to a defective CCR7 signal transduction. To study whether SDC4 may also be qualified as a target for therapeutic interventions, we induced an asthma phenotype first and treated mice with an anti-SDC4 antibody thereafter. This antibody inhibits SDC4 multimerization and SDC4 signalling [14] but will not necessarily affect the expression of the molecule. Interestingly, we observed not only a decreased asthma phenotype after anti-SDC4 treatment, but also the effect on OVA-specific IgE serum levels and Th2 cytokine production was even more distinct in this therapeutic approach than SDC4 inhibition prior to antigen sensitization. This may be due to a different response to the inhibition of SDC4 function related to the time of application considering steady-state DCs versus recruited DCs migrating into already inflamed lung tissue [33] . On the other hand, this might also indicate a role of SDC4 for the function of other cell types. Indeed, activation-dependent upregulation of SDC4 was found in both, DCs and T cells [6] , [8] . It has been shown that depletion of SDC4 + T cells suppressed CHS, an activated T-cell-driven disease [4] . These SDC4 + cells were mainly effector memory T cells comparable to the lung CD4 + SDC4 + T cells we detected in our asthma model, although SDC4 expression is not limited to Th2 cells but detectable on all activated T cells ( Supplementary Fig. 1 ). We further found a reduced CD4 + T-cell proliferation and Th2 cytokine production in antigen-stimulated cell cultures using isolated CD4 + T cells from mediastinal lymph nodes of anti-SDC4-treated BALB/c mice. However, these effects were not caused by a suppression of effector T-cell function through a primary interaction of the antibody with T cells, but were rather a result of the disturbed DC migration leading to a reduced number of activated antigen-specific T cells. In contrast to the CHS suppression by SDC4 + T-cell depletion [4] , in our study the anti-SCD4 Ab did neither deplete SDC4 + T cells nor DCs. Moreover, we could not detect any direct effects of anti-SDC4 Ab on T-cell proliferation or cytokine production after OVA stimulation of DCs co-cultured with T cells containing a transgenic receptor to recognize OVA. However, there might be a microenvironment effect in vivo , which we did not address with our current approach, for example, suboptimal T-cell activation conditions. Thus, the role of T cells cannot be excluded. SDC4 is not only expressed on DCs and T cells but also on other cell types, for example, B cells or eosinophils [9] , [22] . Whereas a large fraction of B cells in the mediastinal lymph nodes express SDC4 in our asthma model ( Fig. 7a ), there was only a very small number of eosinophils in the lung that express SDC4 (<4%, Supplementary Fig. 2 ). Although anti-SDC Ab treatment had neither a direct effect on B-cell activation nor on antibody production, we found a reduced CCL19-directed migration. However, to which extent this decreased B-cell migration into the lymph nodes might contribute to our observed anti-SDC4 Ab effect is not clear yet and has to be further elucidated. Moreover, we cannot exclude that other cell types might be mediating the asthma-reducing effects of SDC4 blockade because of the ubiquitously expression pattern of this molecule. In summary, our results suggest that the primary mode of action of the impaired SDC4 signalling leading to a reduced asthma phenotype is the disturbed DC migration. This applies also for the anti-SDC4 effect during an ongoing immune response, since it is known that DCs play a crucial role in both the initiation and maintenance of allergic airway inflammation [34] . Antigen-loaded APCs seem to be an interesting target for a treatment against allergic immune responses, because they control both the inflammatory and the allergen-specific humoral response [35] . Moreover, inhibition at an early stage of the immune cascade would also suppress the development of memory T and B cells. However, the use of antibodies such as anti-SDC4 to modulate the allergic immune response should require a number of rigorous criteria. The target molecule should be cell specific, expressed at best only in the induction and effector phases of the allergic immune response and in a defined window [35] . Therefore, SDC4 appears not to be an optimal target since it is ubiquitously expressed [6] , [7] . A systemic continuous suppression of SDC4 will likely negatively affect other SDC4-mediated physiological effects with potentially severe undesired consequences. On the other hand, the antibody used inhibits only SDC4 signalling; other functions such as cytokine sequestration remained unaffected. In conclusion, our findings show for the first time that SDC4 plays a crucial role in the development of allergic immune responses. The data also suggest that strategies to inhibit SDC4 might represent a therapeutic option during Th2 cell-mediated allergic inflammatory responses. Mice Female BALB/cByJ and C57BL/6 mice (both 6–8 weeks of age) were obtained from the Elevage Janvier Laboratory (Le Genest St Isle, France). SDC4 −/− mice (backcrossed for 10 generations on C57BL/6 mice) [13] were kindly provided by Sarah Wilcox-Adelman (Boston Biomedical Research Institute, Boston, USA). All animal experiments were performed according to institutional and state guidelines. The Committee on Animal Welfare of Saxony approved animal protocols used in this study. Immunization and antibody treatments SDC4 −/− and WT mice were immunized with OVA (20 μg, Sigma-Aldrich, Steinheim, Germany) adsorbed to 2 mg of an aqueous solution of aluminium hydroxide and magnesium hydroxide (ImjectAlum, Perbio Science, Bonn, Germany) intraperitoneally (i.p.) on days 1 and 14 followed by 20 μg OVA in 40 μl normal saline given i.n. on days 14–16 and 21–23. Control mice received i.p. injections of alum alone and normal saline i.n. AHR was measured at day 24 and mice were killed on day 25. To inhibit SDC4 function, we used a polyclonal antibody against SDC4 ectodomain (200 μg) [14] or nonspecific IgG Abs were applied into BALB/c mice i.p. on days 0 and 13 one day before OVA immunization, respectively. In another protocol mice were immunized with OVA on days 1 followed by OVA i.n. on days 14–16. Control mice received Alum i.p. and normal saline i.n. Anti-SDC4 pAb or control Ab was injected i.p. on days 18 and 22 after the asthma phenotype was already established. Intranasal OVA challenge was repeated on days 21–23 and AHR was measured on day 24. Mice were killed at the following day. Measurement of airway responsiveness Lung resistance ( R L ) was measured by invasive plethysmography (EMKA TECHNOLOGIES, Paris, France) in response to inhaled methacholine (Sigma-Aldrich). Therefore, mice were anesthetized (100 mg kg −1 ketamine and 10 mg kg −1 xylazine, Bayer, Leverkusen, Germany), intubated and mechanically ventilated at a tidal volume of 0.2 ml and a frequency of 150 breath per min. Baseline R L and responses to aerosolized saline (0.9% NaCl) were measured first, followed by responses to increasing doses (2.5 to 40 mg ml −1 ) of aerosolized methacholine. Collection of bronchoalveolar lavage fluid Animals were killed by CO 2 asphyxiation 1 day after the last airway AHR measurement. The trachea was cannulated and the right lung was lavaged three times with 400 μl NaCl 0.9%. Cells in the lavage fluid were counted using a haemocytometer, and BAL cell differentials were determined on slide preparations stained with Diffquick (Medion Diagnostics AG, Düdingen, CH) on blinded samples by an independent investigator. At least 100 cells were differentiated into eosinophils, macrophages, lymphocytes and neutrophils by light microscopy based on conventional morphologic criteria. Lung histology and quantification of inflammation Left lung was fixed in 10% formalin and stained with H&E (MERCK, Darmstadt, Germany). For objective evaluation and quantification of the degree of pulmonary inflammation, lung sections were scanned with a digital camera (Visitron systems, USA, five shots per lung) and analysed with HistoClick-Software based on morphometric image analysis developed in our laboratory [15] , [16] . The degree of inflammation is expressed as the number of pixels that correlate to the stained cells of interest. IgE and IgG 1 assay OVA-specific IgE and IgG 1 serum levels were measured by a sandwich enzyme-linked immunosorbent assay according to a standard protocol [15] , [16] . Briefly, 96-well microtiter plates (Nunc, Roskilde, Denmark) were coated overnight with 10 μg ml −1 OVA diluted in bicarbonate buffer (pH 9.6). After washing and blocking plates, samples were incubated for 2 h. Subsequently, 96-well plates were washed and HRP-conjugated goat-anti-mouse-IgE antibody (Bethyl Laboratories, Montgomery, Texas, USA) was added. Tetramethylbenzidine was used as substrate and the optical density was determined at 450 nm using a Bio-Rad microplate reader (Bio-Rad, Munich, Germany). The titre was calculated by logarithmical regression as the reciprocal dilution of the sera, where the extinction was twofold the background extinction. Cytokine production Splenocytes or mediastinal lymph node cells (5 × 10 6 cells per ml per well) were isolated and restimulated in vitro with 200 μg ml −1 OVA in culture medium (RPMI medium supplemented with 10% FCS, 100 U ml −1 penicilin and 100 μg ml −1 streptomycin) 1 day after the airway function test. Cytokines were measured in supernatants from restimulated spleen or lymph node cells after 3 days using DuoSet ELISA kits (R&D Systems, Minneapolis, USA) according to the manufacturer’s instructions [15] , [16] . Transfer of murine bone-marrow-derived DCs Bone marrow cells were collected from naive WT or SDC4 −/− mice, depleted of red blood cells using ammonium chloride and grown in RPMI medium containing 10% FCS and 20 ng ml −1 recombinant murine granulocyte–macrophage colony-stimulating factor rmGM-CSF for 7 days. Murine CD11c + cells were separated by using magnetic cell sorting systems and CD11c Microbeads (Milteny Biotec, Bergisch Gladbach, Germany). To induce DC maturation, cultures were treated with LPS (1 μg ml −1 , Sigma-Aldrich) for 24 h at day 7. Immunization by intrapulmonal transfer of OVA-pulsed DCs was done as described in refs 36 , 37 . Here, BMDC (2 × 10 6 cells in 80 μl PBS) from SDC4 −/− or WT mice pulsed with OVA (200 μg ml −1 , 24 h) were adoptively transferred into the trachea in anesthetized naive SDC4 −/− or WT mice. From day 10 onwards, mice were challenged i.n. with OVA for 3 consecutive days and killed on day 14 (ref. 16 ). Flow cytometric analysis Cells were measured on BD FACS Canto II (BD Biosciences Pharmingen, Heidelberg, Germany) and experiments were analysed with FACS DIVA and FlowJo software. Dead cells were excluded from analysis by staining with fixable viability dye eFluor 450 (eBioscience). The following isotype controls and anti-murine antibodies were used at 1:50 dilution and purchased from BD rat IgG1-PE (R3-34), CD4-FITC (GK1.5), CD19-PerCP-Cy5.5 (1D3), CD80-PE (16-10A1), CD86-PE (GL1), Syndecan-4-PE (KY/8.2) and ICAM-1-PE (3E2). Rat IgG1-A647 (RTK2071), rat IgG1-PE-Cy7 (RTK2071), CD25-PE-Cy7 (PC61), CD44-APC (IM7), CD45RB-FITC (C363-16A), CD62L-APC (MEL-14), CD69-PE-Cy7 (H1.2F3) and IL-4-A647 (11B11) were from BioLegend. CD11b-FITC (M1/70), CD11c-APC (N418), ICOS-PE (7E.17G9) and IFN-g-APC (XMG1.2) were from eBioscience. Siglec-F-APC (ES22-10D8) and CCR7-Biotin (4B12) were from Miltenyi. Cell surface staining was performed using directly conjugated antibodies and fixed in Cytofix/Cytoperm (BD Biosciences). To analyse the motility of OVA-pulsed DCs into the lymph nodes, bone-marrow-derived DCs from SDC4 −/− or WT mice were pulsed with OVA-Alexa 647 (200 μg ml −1 , Invitrogen, Darmstadt, Germany), stained with CFDA (10 ng, Invitrogen) and 2 × 10 6 cells were adoptively transferred into the trachea in anesthetized mice. Mediastinal lymph nodes were isolated on day 5 and CD11c + CFDA + OVA-Alexa 647 + cells were detected by flow cytometric analysis. To characterize T cells, the lung of OVA-sensitized mice was perfused via the left ventricle with PBS. DNAse- and collagenase-digested lung tissue was strained through a cell strainer (BD Falcon, Germany), lung leucocytes were isolated on Percoll gradient and stained for CD4 + T cells. Ex vivo proliferation and cytokine production BALB/c mice were immunized with OVA (20 μg) i.p. on day 1 followed by i.p. injection of anti-SDC4 pAb or control Ab on days 3 and 7. Mice were challenged i.n. with OVA on days 6–8. The following day, CD4 + T cells from mediastinal lymph nodes were isolated by magnetic cell sorting (CD4 + T-cell isolation kit, Miltenyi). In total, 1 × 10 6 CD4 + T cells were cultured with 2.5 × 10 6 irradiated splenocytes from BALB/c mice (as a source for APCs), stained with CFDA (10 ng) and restimulated with OVA. After 3 days, CDFA fluorescence intensity of CD4 + cells was analysed by flow cytometry and cytokine production was measured in the cell culture supernatant. In vitro proliferation CD4 + T cell from OVA-immunized DO11.10 mice were isolated by magnetic cell sorting and stained with CFDA. In total, 1 × 10 5 T cells were co-cultured with 1.6 × 10 4 OVA-pulsed (200 μg, Sigma) bone-marrow-derived DCs in 96-well tissue culture plates in the presence of IgG or anti-SDC4 antibody. After 4 days of culture, T-cell proliferation was analysed by flow cytometry and cytokine production was measured in the cell culture supernatant. Migration assays To induce maturation, murine BMDCs were treated overnight with LPS (1 μg ml −1 ), while murine with CD19-Microbeads separated B cells from spleens were activated with anti-CD40 (10 μg ml −1 , clone 1C10, eBioscience). Mature cells (1.5 × 10 5 ) were added to upper wells of 5-μm pore, polycarbonate 24-well tissue culture inserts (Costar, Cambridge, USA) in 100 μl, with 600 μl chemokine (100 ng ml −1 CCL19 or CCL21) or medium in the bottom wells. All migration assays were conducted in RPMI with 1% FCS (murine B cells) or 5% FCS (murine DCs) in 5% CO 2 for 3 h at 37 °C. Migrated cells recovered from each lower well were counted with continuous flow for 90 s at a flow cytometer. Co-immunoprecipitation and western blot HEK293 cells (CRL-1573; American Type Culture Collection, Rockville, MD) were transfected using Lipofectamine 2000 (Invitrogen) with a SDC4-flag construct. The next day the cells were incubated for 2 h with 200 ng ml −1 CCL21 (BioLegend), cells were lysed and proteins that had formed a complex with the chemokine were isolated using Anti-FLAGM2 Magnetic Beads (Sigma-Aldrich). Eluted proteins were separated on a 4–15% precast SDS–polyacrylamide gel electrophoresis, transferred to a polyvinylidene difluoride membrane and the blocking anti-SDC4 antibody was used to detect SDC4. CCL21 was detected using human CCL21/6Ckine Antibody (R&D). Non-transfected HEK cells incubated with CCL21 served as negative control. Recombinant CCL21 served as a positive control. Images have been cropped for presentation. Full-size images are presented in Supplementary Fig. 3 . Statistical analysis Student’s unpaired t -test was used to determine the statistical significance of differences between two groups. One-way analysis of variance and Bonferroni’s multiple comparison tests were used when >2 groups were compared. P values of <0.05 were considered significant. How to cite this article: Polte, T. et al . Critical role for syndecan-4 in dendritic cell migration during development of allergic airway inflammation. Nat. Commun. 6:7554 doi: 10.1038/ncomms8554 (2015).